Degradable lipid nanoparticles with predictablein vivosiRNA delivery activity One of the most significant challenges in the development of clinically viable delivery systems for RNA interference therapeutics is to understand how molecular structures influence delivery efficacy. Here, we have synthesized 1,400 degradable lipidoids and evaluate their transfection ability and structure–function activity. We show that lipidoid nanoparticles mediate potent gene knockdown in hepatocytes and immune cell populations on IV administration to mice (siRNA EC 50 values as low as 0.01 mg kg −1 ). We identify four necessary and sufficient structural and pKa criteria that robustly predict the ability of nanoparticles to mediate greater than 95% protein silencing in vivo . Because these efficacy criteria can be dictated through chemical design, this discovery could eliminate our dependence on time-consuming and expensive cell culture assays and animal testing. Herein, we identify promising degradable lipidoids and describe new design criteria that reliably predict in vivo siRNA delivery efficacy without any prior biological testing. The development of drug delivery systems often involves extensive characterization and in vitro testing before the conduct of preclinical studies in rodent or higher order animal models. Unfortunately, progress towards the clinic has been hindered because in vitro results generally do not correlate well with in vivo data [1] , [2] , [3] . This has been particularly true for RNA interference therapeutics (RNAi) [4] . While the past decade has seen an exponential increase in the number of in vitro short interfering RNA (siRNA) delivery studies, very few materials have been reported to mediate potent gene silencing in vivo [5] , [6] , [7] , [8] , and only a handful are being tested in clinical trials [9] . One major challenge in the development of suitable delivery systems is the identification of delivery vehicle chemistries with safety and efficacy characteristics that support a sufficiently broad therapeutic index for chronic indications. This requirement for any kind of RNAi therapeutic stems from the transient nature of gene silencing effects (typically on the order of several days to several weeks in vivo ) and the subsequent need for sustained, repeated siRNA dosing over the course of treatment [10] , [11] . Unfortunately, improvements in delivery vehicle potency do not always result in an enlargement of the therapeutic index due to reductions in tolerated dose levels. In recent years, considerable progress has been made in regards to potency [6] , [12] , but has generally been done so using non-hydrolysable materials. Several challenges associated with delivery vehicle toxicity, degradability and potential for immune stimulation remain [13] , [14] , [15] . With this motivation in mind, we sought to identify degradable materials that enable potent silencing in vivo without causing off-target toxicities (for example, immune system stimulation, necrosis, hepatocellular injury). At the same time, we were interested in the establishment of predictive structure–function relationships that would potentially eliminate the need for costly and time-consuming in vitro screening procedures. One approach towards these dual objectives is the high-throughput screening of libraries of compounds, which can yield large quantities of structure–activity data while significantly increasing the probability of identifying potent delivery compounds [16] , [17] , [18] . Herein, we describe the discovery of several lipid nanoparticles (LNPs) that facilitate high levels of gene silencing in multiple cell subtypes in mice, including hepatocytes, monocytes, macrophages and dendritic cells. Furthermore, we establish a set of four ‘efficacy criteria’ that robustly predict the ability of LNPs to efficiently deliver siRNA without any a priori biological testing. Lipidoid synthesis and nanoparticle formulation In order to develop efficacious, degradable nanoparticles for siRNA delivery while conducting structure–function analysis, we first employed Michael addition chemistry to rapidly synthesize a structurally diverse library of 1,400 lipid-like materials, termed ‘lipidoids’ ( Fig. 1a ). Two-hundred and eighty commercially available alkyl-amines were reacted combinatorially with five alkyl-acrylates of 10–14 carbon chain tail length to form lipidoids consisting of a polar, ionizable core surrounded by hydrophobic carbon tails ( Fig. 1b and Supplementary Fig. 1 ). Although 250 of these materials had been synthesized as part of an earlier study [16] , they have been included here in order to bolster our data set in an effort to develop structure–function relationships. We chose to work with alkyl-acrylate tails of intermediate length, as previous studies indicated that shorter tails often lack efficacy while longer tails may cause insolubility during the nanoparticle formulation process [12] , [16] . These acrylate-based lipidoids also contain hydrolysable ester moieties, functional groups which are commonly incorporated into delivery vehicles to promote physiological degradation [19] , [20] , [21] . Proton NMR analysis indicated that a representative lipidoid, 304O 13 , degraded to the anticipated alkyl-alcohol product under hydrolytic conditions ( Supplementary Figs 2 and 3 ). Conditions were chosen to facilitate the clear observation of degradation products by NMR. It should be noted that, in vivo , lipidoids would be expected to degrade in the presence of liver-produced enzymes, particularly esterases [22] , [23] . 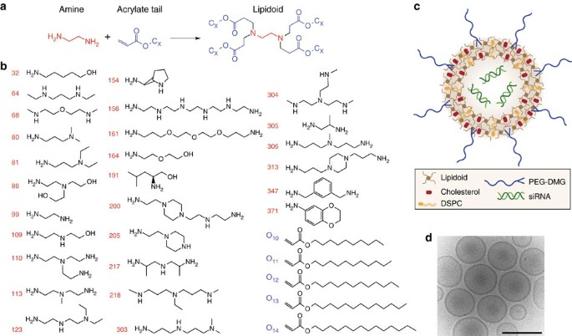Figure 1: Lipidoid nanoparticle synthesis. A library of 1,400 biodegradable lipidoids was synthesized combinatorially through the (a) conjugate addition of alkyl-amines (in red) to alkyl-acrylate tails (in blue). (b) A subset of the 280 amines used (complete listing inSupplementary Fig. 1) are shown here. (c) Lipidoids were formulated with cholesterol, the phospholipid DSPC, PEG2000-DMG and siRNA to form nanoparticles. (d) A cryo-transmission electron microscopy image of lipidoid nanoparticles. Scale bar, 100 nm. Figure 1: Lipidoid nanoparticle synthesis. A library of 1,400 biodegradable lipidoids was synthesized combinatorially through the ( a ) conjugate addition of alkyl-amines (in red) to alkyl-acrylate tails (in blue). ( b ) A subset of the 280 amines used (complete listing in Supplementary Fig. 1 ) are shown here. ( c ) Lipidoids were formulated with cholesterol, the phospholipid DSPC, PEG2000-DMG and siRNA to form nanoparticles. ( d ) A cryo-transmission electron microscopy image of lipidoid nanoparticles. Scale bar, 100 nm. Full size image In vitro screening of LNPs for siRNA delivery Before testing the transfection ability of lipidoids, they were first formulated into LNPs containing siRNA and the helper lipids cholesterol, 1,2-distearoyl- sn -glycero-3-phosphocholine (DSPC) and PEG2000-DMG ( Fig. 1c ). Depending on the lipidoid, these particles had an average diameter of 60–120 nm. A representative cryo-transmission electron microscopy image is shown in Fig. 1d . Delivery potential was assessed by applying LNPs to HeLa cells that stably expressed two reporter luciferase proteins: firefly and Renilla . Firefly and Renilla luciferases served as the target and control genes, respectively. Any delivery materials that caused reductions in Renilla luciferase activity, which suggested the presence of either cytotoxicity or off-targeting effects, were not considered further. Relative luciferase activity, which is the normalized value of firefly activity, is shown in Fig. 2a after treatment with each LNP at an siRNA concentration of 40 nM. Of the 1,400 members of the lipidoid library, 82 mediated firefly luciferase silencing of >50% (red data points). 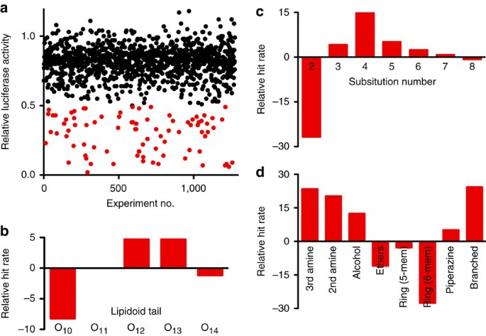Figure 2:In vitrosiRNA delivery activity of lipidoid nanoparticles. (a) Relative luciferase activity values (normalized to controls) are shown for 1,400 lipidoids. ~7% of the library induced >50% gene silencing (shown in red). s.d. (not depicted for the sake of clarity) averaged 0.05 (n=4). (b) The tail length, (c) tail substitution number and (d) alkyl-amine composition influencedin vitroactivity. Structural features that were common among efficacious materials had positive Relative Hit Rate values. Figure 2: In vitro siRNA delivery activity of lipidoid nanoparticles. ( a ) Relative luciferase activity values (normalized to controls) are shown for 1,400 lipidoids. ~7% of the library induced >50% gene silencing (shown in red). s.d. (not depicted for the sake of clarity) averaged 0.05 ( n =4). ( b ) The tail length, ( c ) tail substitution number and ( d ) alkyl-amine composition influenced in vitro activity. Structural features that were common among efficacious materials had positive Relative Hit Rate values. Full size image In order to extract structure–function information from the in vitro data, we asked whether various structural properties were more or less common within the group of efficacious lipidoids (red data points) compared with the bulk library. Figure 2b examines the importance of tail length on transfection. Because there were five tails used in this library, each tail length made up 20% of the library. Of the LNPs that were effective in vitro , however, only 12% contained an O 10 tail. Relative hit rate (the y axis value) was calculated as (percentage in the group with >50% silencing)−(percentage in the library). Therefore, the relative hit rate for O 10 is 12−20%=−8%, indicating that an O 10 tail was significantly underrepresented among materials with transfection potential. On the other hand, O 12 and O 13 tails were overrepresented in the efficacious group compared with the library at large, suggesting that such tail lengths are associated with efficacious lipidoids. Figure 2c indicates that potent lipidoids were synthesized from alkyl-amines with three or more substitution sites. The effect of various functional groups within the alkyl-amine is analysed in Fig. 2d . In general, the presence of tertiary and secondary amines, alcohols and branched or linear chains conferred efficacy, while ethers and rings did not. Piperazine rings, however, were an exception, and generally produced efficacious materials (likely because they contained tertiary amines). It has been repeatedly suggested in the literature that the presence of amines confers increased buffering capacity and endosomal escape [24] . The reasons for the other trends are currently unclear, although there have been other reports of efficacious siRNA delivery materials that contain alcohols [12] and heavy branching [25] , [26] . Top LNPs mediate potent gene silencing in vivo Previous studies have indicated that materials conferring >50% luciferase silencing activity in cell culture have the potential to mediate siRNA delivery in vivo [4] . As such, the lipidoids shown in red in Fig. 2a were analysed for the ability to deliver siRNA in mice. We chose to target Factor VII, a blood clotting factor produced specifically in hepatocytes. Factor VII is well-suited for such studies, as it has a short half-life and can be readily quantified from a small serum sample [6] , [16] , [27] . In these experiments, LNPs containing anti-Factor VII siRNA were injected intravenously into mice, and Factor VII activity levels were quantified 2 days post injection. Fifteen of the 96 lipidoids analysed in vivo mediated very high levels of knockdown of Factor VII protein levels at an siRNA dose of 5 mg kg −1 (red data points, Fig. 3a ). For these top LNP candidates, control experiments conducted using non-targeting siRNA at 5 mg kg −1 resulted in no FVII knockdown and suggested that reductions in protein activity were not due to off-target effects. Silencing for the top candidates was dose dependent ( Supplementary Fig. 4 ), with EC 50 values ranging from 0.05 to 2 mg kg −1 ( Fig. 3b ) when LNPs were formulated at a lipidoid: cholesterol: DSPC: polyethylene glycol (PEG) standard testing molar ratio of 50:38.5:10:1.5, chosen based on the formulation optimization of previously studied lipidoid nanoparticles [12] . Importantly, the choice of helper lipids did not affect the relative efficacy of lipidoid compounds. 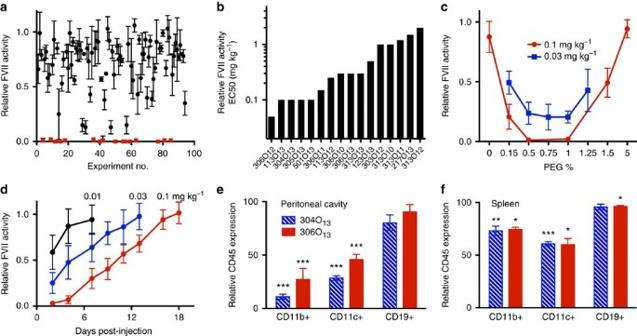Figure 3:In vivosiRNA delivery activity of lipidoid nanoparticles. (a) Of the ~100 lipidoids tested in mice, 15 induced high levels of Factor VII knockdown at a total siRNA dose of 5 mg kg−1(data points in red). (b) The EC50 values of these top 15 lipidoids ranged from 0.05 to 1.5 mg kg−1under standard formulation conditions. (c) The amount of PEG in the LNP formulation had a dramatic effect on efficacy. Data is shown for the lipidoid 304O14, which was optimally formulated with 0.75 mol% PEG. (d) Dose response and Factor VII activity recovery data for the optimized 304O13LNP formulation. (e) 304O13also induced CD45 silencing in monocyte and macrophage (CD11b+) populations in the peritoneal cavity (f) as well as in dendritic cells (CD11c+) in the spleen 3 days post injection. Ineandf, ***, ** and * correspond toP-values <0.0005, 0.005 and 0.05, respectively, by an unpaired student’st-test when comparing with LNPs containing non-targeting siRNA. In all panels, error bars represent s.d. (n=3). Figure 3: In vivo siRNA delivery activity of lipidoid nanoparticles. ( a ) Of the ~100 lipidoids tested in mice, 15 induced high levels of Factor VII knockdown at a total siRNA dose of 5 mg kg −1 (data points in red). ( b ) The EC50 values of these top 15 lipidoids ranged from 0.05 to 1.5 mg kg −1 under standard formulation conditions. ( c ) The amount of PEG in the LNP formulation had a dramatic effect on efficacy. Data is shown for the lipidoid 304O 14 , which was optimally formulated with 0.75 mol% PEG. ( d ) Dose response and Factor VII activity recovery data for the optimized 304O 13 LNP formulation. ( e ) 304O 13 also induced CD45 silencing in monocyte and macrophage (CD11b+) populations in the peritoneal cavity ( f ) as well as in dendritic cells (CD11c+) in the spleen 3 days post injection. In e and f , ***, ** and * correspond to P -values <0.0005, 0.005 and 0.05, respectively, by an unpaired student’s t -test when comparing with LNPs containing non-targeting siRNA. In all panels, error bars represent s.d. ( n =3). Full size image While seeking an optimal molar ratio for the top LNPs (for example, 306O 12 , 113O 13 and 304O 13 ), the PEG molar percentage, in particular, was found to have a dramatic effect on LNP efficacy. Figure 3c shows that, for the lipidoid 304O 13 , there is a very narrow window of PEG % between 0.5 and 1.0 where optimal hepatocellular delivery is achieved. The optimized 304O 13 formulation (PEG%=0.75) has an EC 50 value, 0.01 mg kg −1 , which is a full order of magnitude lower than when using a PEG% of 1.5. Optimized 304O 13 behaved in a dose dependent fashion ( Fig. 3d ), and after a single injection at 0.1 mg kg −1 , Factor VII levels remained suppressed for 18 days. In addition to examining hepatocellular delivery, we also explored the ability of degradable lipidoid materials to deliver siRNA to leukocyte populations in vivo . Specifically, we wondered whether or not chemistries that were effective for hepatocyte delivery might also have utility in white blood cell populations. Immune cells are attractive targets for RNAi therapy, as they have been implicated in various aspects of disease initiation and progression, including inflammation and autoimmune responses [28] , [29] . There have been several previous reports of siRNA delivery to leukocytes, including polyketal microparticle delivery to liver macrophages [30] and lipid nanoparticle delivery to macrophages and monocytes [7] , [31] . It is anticipated that ultimate clinical utility will likely require the use of degradable compounds that can be eliminated from the body. In these experiments, LNPs were formulated with siRNA specific against CD45, which is a tyrosine phosphatase protein found on the surface of all white blood cells [32] . Three days following the intravenous delivery of LNPs in mice, immune cells were harvested from the peritoneal cavity and spleen. Cells were stained with fluorescent antibodies, and CD45 protein silencing was quantified in specific immune cell subsets via flow cytometry analysis. Results were normalized to CD45 levels after delivery of the same LNP containing a non-targeting siRNA. Of the five lipidoid materials evaluated in this model, 304O 13 and 306O 13 mediated the most robust CD45 silencing in immune cells isolated from both the peritoneal cavity and the spleen ( Fig. 3e,f ). CD11b+ and CD11c+ populations (monocyte/macrophages and dendritic cells, respectively) were subject to high levels of knockdown within the peritoneal cavity (up to 90%) and to a lesser degree within the spleen (up to 40%). The lipidoids 306O 12 , 306O 14 and 315O 12 also offered modest CD45 silencing in several immune cell subpopulations ( Supplementary Fig. 5 ). LNP characterization and biodistribution in mice Nanoparticle characterization parameters for three of the top LNP candidates were similar ( Table 1 ). Entrapment of siRNA refers to the percentage of siRNA in solution that is incorporated into the nanoparticle during formulation, as measured by an RNA dye-binding assay [33] . These results are in keeping with a previous finding that efficacious lipidoid nanoparticles often have entrapment values of approximately 75% (ref. 4 ). Zeta potential measurements were conducted under neutral pH conditions. pKa values, which were obtained using a 2-( p -toluidino) naphthalene-6-sulphonic acid (TNS) assay, evaluated the pKa of the nanoparticle surface [34] . The pKa values of top LNP candidates corroborate the results of another study in which surface pKa values in the 6–7 range conveyed efficacy in vivo [35] . Table 1 Characterization parameters for top LNPs. Full size table Several analyses were performed to assess the biodistribution of the lead compound, 304O 13 , in mice. For these experiments, nanoparticles were formulated with Cy5.5-labelled siRNA. Whole-organ IVIS images ( Fig. 4a ) and Odyssey scans ( Fig. 4b ) showed that naked siRNA accumulated in the kidneys at 1 h post injection, suggesting rapid renal clearance. Quantification of IVIS signal indicated that 14, 1 and 71% of naked siRNA signal appeared in the liver, spleen and kidneys, respectively. In contrast, at 1 h post injection, 304O 13 localized primarily within the liver (42%) and spleen (24%), with only 18% distributing to the kidneys. 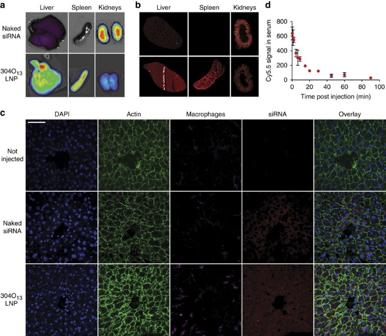Figure 4: Biodistribution images for Cy5.5-labelled siRNA delivered with the lipidoid 304O13. (a) IVIS and (b) Odyssey imaging show that, while naked siRNA is primarily cleared through the kidneys, 304O13mediates accumulation in the liver and spleen. (c) Confocal microscopy of 304O13-treated liver shows siRNA (red) delivery throughout the tissue, including Kupffer cells (magenta) and hepatocytes (nuclei in blue and actin cytoskeleton in green). Three animals were tested per condition for experiments depicted ina–cand the images shown are representative. Scale bar, 50 μm. (d) 304O13LNPs were rapidly eliminated from the bloodstream after tail vein injection. Error bars represent s.d. (n=3). Figure 4: Biodistribution images for Cy5.5-labelled siRNA delivered with the lipidoid 304O 13 . ( a ) IVIS and ( b ) Odyssey imaging show that, while naked siRNA is primarily cleared through the kidneys, 304O 13 mediates accumulation in the liver and spleen. ( c ) Confocal microscopy of 304O 13 -treated liver shows siRNA (red) delivery throughout the tissue, including Kupffer cells (magenta) and hepatocytes (nuclei in blue and actin cytoskeleton in green). Three animals were tested per condition for experiments depicted in a – c and the images shown are representative. Scale bar, 50 μm. ( d ) 304O 13 LNPs were rapidly eliminated from the bloodstream after tail vein injection. Error bars represent s.d. ( n =3). Full size image Given their effectiveness for silencing the hepatocellular target, FVII, we examined how 304O 13 nanoparticles were distributing within the liver. Confocal imaging was performed on liver tissues harvested 1 h post injection and stained with nuclear, actin and macrophage markers ( Fig. 4c ). Images were taken near the central vein in liver lobules (black void near the centre of images). Hepatocytes are outlined in green and macrophages, which appear sporadically, are coloured magenta. Only 304O 13 was able to mediate siRNA accumulation throughout nearly all hepatocellular tissue (in red). Serum clearance kinetics were assessed by measuring Cy5.5 signal in the mouse bloodstream as a function of time ( Fig. 4d ). It should be noted that, while the first blood sample was drawn as quickly as possible (20 s), maximum signal may have occurred even earlier. Half of the material initially detected at 20 s had distributed to tissues by 6 min. At 90 min post injection, only 4% of the signal remained. Safety assessment of lead LNP 304O 13 We conducted a preliminary safety assessment of the lead LNP, 304O 13 , and compared it with a another previously discovered LNP formulation, C12-200 [12] . C12-200 is a five-tailed, lipidoid that has the same EC 50 as 304O 13 (0.01 mg kg −1 ). It also has nearly identical biodistribution properties as 304O 13 (data not shown). It was chosen for comparison purposes because it does not contain any functional groups that are overtly sensitive to hydrolysis. We chose to examine the effect of doses that were at least 100-fold higher than the EC 50 . Serum cytokine levels for both materials were assessed in mice 4h after a 3 mg kg −1 IV bolus injection (total siRNA). The cytokines chosen were expected to reflect an innate immune response either to foreign material [13] or to liver irritation [36] . Interleukin-6, inducible protein-10, keratinocyte chemoattractant and monocyte chemoattractant protein 1 were elevated in the C12-200 group compared with both phosphate-buffered saline (PBS) negative control and 304O 13 groups under these conditions ( Supplementary Fig. 6 ). Clinical chemistry parameters were evaluated for both materials 72 h after a single dose of 3 mg kg −1 and after four, once weekly doses of 3 mg kg −1 each. There were no toxicologically significant increases in albumin, alanine transaminase, aspartate transaminase, alkaline phosphatase, total bilirubin or gamma-glutamyl transferase for either 304O 13 or C12-200 after single or multiple doses ( Supplementary Fig. 7 ). Finally, histological analysis was performed through hematoxylin and eosin staining on sections from the liver, spleen, kidneys and pancreas. In single-dose studies (0, 1, 2, 3, 5, 7.5, 10 mg kg −1 ), liver necrosis was observed in mice administered ≥7.5 mg kg −1 of C12-200 and at 10 mg kg −1 of 304O 13 . Pancreatic inflammation and islet cell enlargement were detected at C12-200 doses ≥2 mg kg −1 . A small amount of apoptosis in splenic red pulp was observed at 10 mg kg −1 for 304O 13 . Multidose studies were also conducted in which mice received four injections of 0.3, 1, 2, 3 or 5 mg kg −1 , once per week for 4 weeks. Liver necrosis and inflammation were observed in mice administered ≥1 mg kg −1 of C12-200. There was no sign of liver toxicity in any of the 304O 13 groups up to 5 mg kg −1 . On the basis of this limited evaluation, the collective data suggest an improved toxicity profile for 304O 13 compared with C12-200 in mice. It should be noted that toxicity testing is material specific, and results for 304O 13 cannot be broadly extended to the other materials in this study without further analysis. Predictive structure–function relationships We closely examined the data from the materials tested in vivo at a total siRNA dose of 5 mg kg −1 for any relationship that may exist between chemistry and delivery ability to the liver. We found three structural properties that had a striking effect on efficacy in vivo ( Fig. 5a ). Of the 96 materials tested in mice, 25 of them contained an O 13 tail (yellow circle), 66 of them had three or more tails (blue circle) and 42 of them had been synthesized from an alkyl-amine that contained at least one tertiary amine (red circle). When a lipidoid possessed all three of these properties (shown by the three-way overlap of circles), it was able to mediate very high levels of Factor VII silencing in the liver 88% of the time. When only one of these properties was removed from a lipidoid, the likelihood of achieving high levels of knockdown dropped significantly to 17–31%. Finally, when a material conformed to only one (or none) of these three structural ‘efficacy criteria’, Factor VII silencing ability was uniformly lost. The presence of tertiary amines in a delivery material are thought to enhance the material’s buffering capacity and ability to induce endosomal escape [37] , [38] , [39] . In this study, tertiary amines exist in a lipidoid either because of those present in the original alkyl amine or those created on conjugation of tails—both are shown here to improve efficacy. The importance of precise tail length is less clear at this time. 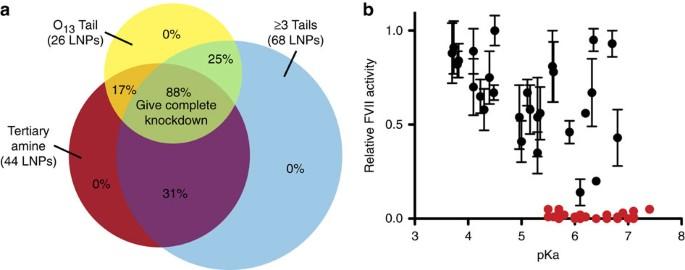Figure 5: Lipidoids showed strong structure–function relationshipsin vivo. (a) Of the 96 LNPs tested for siRNA delivery to hepatocytes in mice, 68 had three or more tails (blue), 44 had a tertiary amine present in the original alkyl-amine (red) and 26 had an O13tail length (yellow). Eighty eight percent of the LNPs exhibiting all three structural ‘efficacy criteria’ (overlap of circles) achieved nearly complete FVII knockdown. The probability of identifying efficacious LNPs decreased precipitously when any of the criteria were not met. (b) pKa values also significantly influenced delivery efficacy to hepatocytesin vivo. All lipidoid nanoparticles capable of mediating nearly complete Factor VII gene silencing had pKa values ≥5.5. Error bars represent s.d. (n=3). Figure 5: Lipidoids showed strong structure–function relationships in vivo . ( a ) Of the 96 LNPs tested for siRNA delivery to hepatocytes in mice, 68 had three or more tails (blue), 44 had a tertiary amine present in the original alkyl-amine (red) and 26 had an O 13 tail length (yellow). Eighty eight percent of the LNPs exhibiting all three structural ‘efficacy criteria’ (overlap of circles) achieved nearly complete FVII knockdown. The probability of identifying efficacious LNPs decreased precipitously when any of the criteria were not met. ( b ) pKa values also significantly influenced delivery efficacy to hepatocytes in vivo . All lipidoid nanoparticles capable of mediating nearly complete Factor VII gene silencing had pKa values ≥5.5. Error bars represent s.d. ( n =3). Full size image Furthermore, we found that the surface pKa of LNPs played an important role in determining in vivo efficacy. Studies have shown that the ability of materials to take on a positive charge with decreasing pH may confer transfection efficacy which would point to pKa as a critical parameter [35] , [40] . Data in Fig. 5b indicate that surface pKa values play a decisive role in this system, with a critical pKa value of approximately 5.5. All materials demonstrating considerable in vivo transfection ability (red data points) had surface pKa values of 5.5 or higher. For values less than 5.5, average efficacy decreased monotonically with pKa. This parameter explains the few materials represented in Fig. 5a that failed to produce significant gene silencing despite having met all three structural efficacy criteria. Therefore, we concluded that lipid nanoparticle efficacy is subject to a fourth criterion, which is that the pKa must meet or exceed 5.5. Notably, the structural criteria can be determined on the basis of structure alone, while the pKa criteria requires only a simple, non-biological assay. Table 2 shows a four-way analysis of the efficacy criteria and confirms the importance of conforming to all four criteria to guarantee high levels of gene silencing in vivo . Table 2 Importance of efficacy criteria on in vivo gene silencing. Full size table Second-generation library confirms efficacy criteria To investigate our ability to predict in vivo siRNA delivery potency without any biological testing, we custom synthesized a small second-generation library of amines ( Fig. 6a ) which, when conjugated to an O 13 tail, produced lipidoids that met the three structural efficacy criteria. As such, we expected a large fraction of this second-generation ‘test’ library to be efficacious in comparison with first generation lipidoids. Once formulated into nanoparticles, we determined that all of the second-generation lipidoids resulted in surface pKa values ≥5.5, except for 509O 13 and 510O 13 . These lipidoids had surface pKa values of 3.7 and 4.1, respectively. Therefore, we hypothesized that all of the 500 series lipidoids, with the exception of 509O 13 and 510O 13 , should have potent siRNA delivery activity in mice. When tested in vivo in the Factor VII model at a dose of 5 mg kg −1 , we found that our predictions were uniformly accurate ( Fig. 6b ). All materials induced greater than 95% silencing, with the exception of 509O 13 and 510O 13 , which each mediated only 10% silencing and are not included in the graph. The dose dependence of gene knockdown was investigated in order to identify highly efficacious materials in addition to those from the first generation library, and EC 50 values were found to vary from 0.05 to 1 mg kg −1 ( Fig. 6c ). Formulation optimization of the best second-generation material, 503O 13 , markedly decreased the EC 50 value to 0.01 mg kg −1 ( Fig. 6d ). Several second-generation materials also facilitated significant CD45 knockdown in monocyte, macrophage, dendritic cell and B-cell populations ( Supplementary Fig. 8 ). At the highest dose tested, 5 mg kg −1 , 500 series LNPs did not cause any reductions in mouse bodyweights, suggesting that these second-generation materials were not acutely toxic ( Supplementary Fig. 9 ). 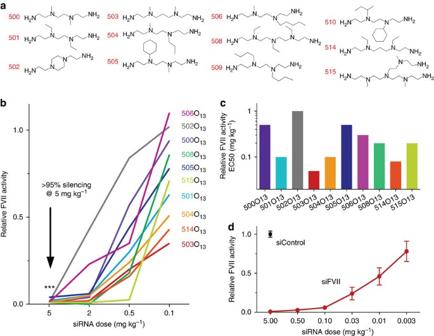Figure 6: A second-generation library confirmed structure–function relationships. Twelve second-generation LNPs were made to meet structural efficacy criteria by first synthesizing custom alkyl-amines shown inaand reacting them with O13tails. (b) All second-generation LNPs meeting structural and pKa criteria abrogated Factor VII activityin vivo(P-values <0.0005 by an unpaired student’st-test) and (c) their EC50s under non-optimized LNP formulating conditions ranged from 0.05 to 1 mg/kg total siRNA. (d) 503O13was the most efficacious LNP on formulation, with an EC50of 0.01 mg kg−1. 503O13encapsulating control siRNA (black data point) did not result in FVII knockdown. Error bars represent s.d. (n=3). There was a statistically significant difference between groups as determined by one-way analysis of variance (F(6,14)=86.69,P<0.0001).Post hoccomparisons using the Tukey HSD test indicated that all tested doses of 503O13resulted in silencing levels that were significantly different than the siControl (P<0.05). Figure 6: A second-generation library confirmed structure–function relationships. Twelve second-generation LNPs were made to meet structural efficacy criteria by first synthesizing custom alkyl-amines shown in a and reacting them with O 13 tails. ( b ) All second-generation LNPs meeting structural and pKa criteria abrogated Factor VII activity in vivo ( P -values <0.0005 by an unpaired student’s t -test) and ( c ) their EC50s under non-optimized LNP formulating conditions ranged from 0.05 to 1 mg/kg total siRNA. ( d ) 503O 13 was the most efficacious LNP on formulation, with an EC 50 of 0.01 mg kg −1 . 503O 13 encapsulating control siRNA (black data point) did not result in FVII knockdown. Error bars represent s.d. ( n =3). There was a statistically significant difference between groups as determined by one-way analysis of variance (F(6,14)=86.69, P <0.0001). Post hoc comparisons using the Tukey HSD test indicated that all tested doses of 503O 13 resulted in silencing levels that were significantly different than the siControl ( P <0.05). Full size image In recent years, it has become increasingly important to consider the degradability of siRNA delivery materials and their potential for immune stimulation. While earlier efforts focused on potency, clinical translation requires materials that are nontoxic enough to allow the repeated delivery that is typically needed for transient RNAi therapy. Part of what has made this so challenging from a research perspective is that potency can be measured via one endpoint, but there are many potential endpoints when evaluating toxicity and immunogenicity. This study has identified a potent lipidoid nanoparticle, 304O 13 , that did not pose preliminary toxicity concerns at doses less than two orders of magnitude above than the EC 50 . In this study, we chose to evaluate cytokine expression and clinical chemical parameters at selected time points post injection and to perform histological analysis on liver sections exposed to LNPs. Such work, although resource intensive, represents a fraction of potential endpoints that may reveal toxicity issues for a particular compound [41] . As such, conclusions regarding the safety profile of 304O 13 or extension to other members of the lipidoid library should be done with caution. The synthesis and biological testing of large libraries of materials, such as the one described in Fig. 1 , offer several advantages in the development of delivery systems. First, the probability of discovering a potent delivery vehicle is significantly increased. Second, traditional drug delivery bias towards certain chemistries can be avoided if sufficient diversity is incorporated into the library. Third, and perhaps most importantly, the large quantity of screening results can be used to establish structure–function relationships that can inform the development of second-generation libraries of increasingly efficacious materials. It is rare that structure–function studies reveal trends as strong as those demonstrated in Fig. 5 and Table 2 . Specifically, lipidoids synthesized from O 13 tails and alkyl-amines containing at least one tertiary amine and at least three substitution sites had a high probability of facilitating potent gene silencing in mice. If a simple, non-biological assay is performed to assess the pKa, LNPs with pKa values less than or equal to 5.4 can be ruled out. This nearly ensures high levels of in vivo knockdown. Of the four criteria, pKa appears to be the most influential in determining in vivo efficacy in this system. It is the only criterion that, when not met, abolishes the ability of an LNP to facilitate high levels of gene silencing. In summary, we have synthesized and tested a library of over 1,400 lipid-like compounds for siRNA delivery in an attempt to develop robust structure–function relationships that can inform the future work of drug delivery scientists. In the process, we identified numerous degradable lipidoid formulations capable of mediating very potent gene silencing in multiple biological targets (including hepatocytes and immune cells) in mice after IV administration. One of the top formulations offered an improved toxicity profile in comparison with a lead non-degradable lipidoid formulation, and materials possessing potential clinical utility are presently being evaluated in higher order animal models. Given the general difficulty of establishing structure–activity relationships in vivo , we were surprised to discover a set of four efficacy criteria (three structural and one pKa) that robustly predict in vivo siRNA delivery potency. Importantly, these material design principles are able to predict in vivo activity without any prior biological testing. In the context of future work, these new findings may hasten delivery material development by reducing our dependence on time-consuming and expensive cell culture and animal testing while underscoring a need for synthetic chemistry innovation. Lipidoid synthesis Lipidoids were synthesized through the addition of alkyl-acrylates to amines. Amines were purchased from Sigma Aldrich (St Louis, MO), Alfa Aesar, Acros Organics and CHESS Organics. Briefly, 500 series amines were synthesized by reacting secondary amines with sodium cyanide to form a nitriles, which were reduced to the primary amine products using lithium aluminium hydride [42] . Acrylates were purchased from Scientific Polymer Products (Ontario, NY) and Hampford Research, Inc. (Stratford, CT). To synthesize lipidoids, amines were combined with acrylates stoichiometrically in a glass scintillation vial and were stirred at 90 °C for 3 days. In vitro experiments were conducted with crude materials while i n vivo experiments were performed with lipidoids that were either crude or purified via a Teledyne Isco Chromatography system (Lincoln, NE). Details of chemical characterization of a representative selection of compounds can be found in Supplementary Note 1 . Lipidoid hydrolysis To a 25 ml round bottom flask was added 304O 13 (0.250 g, 0.263 mmol, 1 equiv). For acidic hydrolysis, 10 ml of a solution of 6 N HCl was added to the flask to afford a cloudy heterogeneous solution. The reaction was heated to reflux to afford a clear, homogeneous solution and was stirred at reflux for 24 h. For basic hydrolysis, 10 ml of a solution of KOH in EtOH/H 2 O (solution=5.61 g KOH in 47.5 ml EtOH w/2.5 ml distilled H 2 O) was added to the flask to afford a clear colourless solution. The reaction was heated to reflux and stirred for 41 h. Both acidic and basic reactions were cooled to room temperature and thin-layer chromatography analysis showed the presence of tridecanol (17.5% EtOAC/Hexanes) and the consumption of 304O 13 . Reactions were concentrated to dryness under reduced pressure and diluted with CDCl 3 . The basic reaction was filtered to remove excess KOH. Proton NMR analysis was performed in CDCl 3 . Proton nuclear magnetic resonance spectra were recorded with a Bruker Avance 400 spectrometer, are depicted in parts per million on the δ scale, and are referenced from the residual protium in the NMR solvent (CDCl 3 : δ 7.26 (CHCl 3 ). Formulation of LNPs Lipidoids were formulated into nanoparticles for all applications. Nanoparticles were formed by mixing lipidoids, cholesterol (Sigma Aldrich), DSPC (Avanti Polar Lipids, Alabaster, AL) and mPEG2000-DMG (MW 2660, gift from Alnylam Pharmaceuticals, Cambridge, MA) at a molar ratio of 50:38.5:(11.5−X):X in a solution of 90% ethanol and 10% 10 mM sodium citrate (by volume). An siRNA solution was prepared by diluting siRNA in 10 mM sodium citrate such that the final weight ratio of lipidoid: siRNA was between 5:1 and 10:1, depending on the experiment. Equal volumes of lipid solution and siRNA solution were rapidly mixed together using either a microfluidic device [43] or by pipet to form nanoparticles. Particles were diluted in PBS, Invitrogen, Carlsbad, CA and then dialysed against PBS for 90 min in 3,500 MWCO cassettes (Pierce/Thermo Scientific, Rockford, IL). In vitro transfection of cell lines with LNPs HeLa cells (American Type Culture Collection, Manassas, VA) stably modified to express both firefly and Renilla luciferase were maintained at 37 °C in high glucose Dulbecco’s Modified Eagles Medium without phenol red (Invitrogen) supplemented with 10% fetal bovine serum (Invitrogen). 12–16 h before transfection, cells were seeded in white 96-well plates at a density of 15,000 cells per well. Cells were transfected with a 40 nM concentration of anti-firefly luciferase siRNA (Dharmacon, Lafayette, CO) that had been formulated with lipidoids into nanoparticles. Firefly luciferase silencing was assessed with a Dual-Glo Luciferase Assay kit (Promega, Madison, WI). Renilla luciferase activity served as a control. In vivo gene silencing All animal experiments were conducted using institutionally-approved protocols (IACUC). Female C57BL/6 mice at least 6 weeks of age (Charles River Laboratories, Wilmington, MA) received lateral tail vein injections of PBS (negative control) or lipidoid nanoparticles containing either non-targeting siRNA (negative control) or anti-Factor VII siRNA diluted in PBS at a volume of 0.01 ml g −1 . The sequence of the siFVII, provided by Alnylam Pharmaceuticals, was: sense: 5′-GGAucAucucAAGucuuAcT*T-3′; antisense: 5′-GuAAGAcuuGAGAuGAuccT*T-3′,where 2′-fluoro-modified nucleotides are in lower case and phosphorothioate linkages are represented by asterisks. Two days post injection, a 100 μl blood sample was obtained from mice, and serum levels of Factor VII were analysed using a Biophen FVII assay kit as described previously (Aniara Corporation, Mason, OH) [6] . Biodistribution and immunostaining Female C57BL/6 mice received tail vein injections LNPs containing siRNA that had been labelled with Cy5.5 on the 5′-end of the sense strand (provided by Alnylam Pharmaceuticals). Animals were dosed at 1 mg/kg of siRNA and volume of 0.01 ml g −1 . At 1 h post injection, mice were euthanized and organs were removed. Body-wide biodistribution was assessed by imaging whole, unprocessed organs with an IVIS Spectrum system (Caliper Life Sciences, Hopkinton, MA) at excitation and emission wavelengths of 675 and 720 nm, respectively. For Odyssey and confocal imaging, organs were snap frozen on dry ice and embedded in optimal cutting temperature compound (Life Technologies, Grand Island, NY). Cryostat sections were cut and collected on superfrost plus treated slides. Prepared frozen sections where kept at −20 °C until needed. Odyssey imaging was conducted on 20-μm-thick cryosections of tissue at a resolution of 21 μm [44] . For confocal imaging, liver tissue was cryosectioned (12 μm) and fixed using 4% paraformaldehyde at room temperature for 30 min. All solutions were prepared in PBS. Sections were washed two times with PBS, permeabilized for 30 min with 0.1% Triton X100 and blocked for 1 h with 5% normal goat serum. Sections then incubated for 1 h in an immunostaining cocktail solution consisting of 4′,6-diamidino-2-phenylindole (3 μM), Alexa Fluor 488 conjugated anti-mouse F4/80 (1:200 dilution, BioLegend, San Diego, CA), Alexa Fluor 555 Phalloidin (1:200 dilution, Life Technologies) and 5% normal goat serum. Slides were washed three times with 0.1% Tween 20 and mounted using ProLong Gold Antifade (Life Technologies). Sections were imaged using an LSM 700 point scanning confocal microscope (Carl Zeiss, Inc, Jena Germany) equipped with a × 40 oil immersion objective. Blood clearance Blood clearance experiments were conducted by injecting LNPs containing Cy5.5-labelled siRNA at an siRNA dose of 0.5 mg kg −1 . Blood samples were collected as a function of time via the retroorbital vein, with the exception of final time points, which were collected via cardiac puncture. Serum, obtained by centrifugation, was diluted 1:30 in PBS and imaged and quantified using an Odyssey CLx imaging system (LI-COR Biosciences, Lincoln, NE). Histology Animals that had received various doses of either 304O 13 or C12-200 LNPs were killed, and their organs were collected immediately. Organs were fixed overnight in 4% paraformaldehyde and transferred to 70% ethanol before paraffin embedding, sectioning and hematoxylin and eosin staining. Serum chemistry and cytokine analysis Post killing, cardiac sticks were immediately performed on animals that had been dosed with either 304O 13 or C12-200 LNPs. A dose of 3 mg kg −1 was used for cytokine and serum chemistry experiments. Blood was centrifuged in serum separator tubes at 5,000 r.p.m. for 10 min before analysis. Serum chemistry was evaluated on a Beckman Olympus AU400 Serum Chemistry Analyzer. Cytokines were analysed using Bio-Plex Pro Mouse Cytokine 23-Plex Assay kits (Luminex Corporation, Austin, TX) on the Bio-Plex 200 system, according to the manufacturer’s instructions. Nanoparticle characterization LNPs were diluted to an siRNA concentration of ~4 μg ml −1 in PBS buffer, pH 7.4. siRNA entrapment efficiency was determined using the Quant-iT RiboGreen RNA assay (Invitrogen). Particle sizes were measured with a ZETAPals analyzer (Brookhaven Instruments, Holtsville, NY). Sizes reported are the average effective diameter of each LNP. Zeta potential measurements were acquired on a Zetasizer Nano ZS (Malvern, Westborough, MA), and reported values were the average of 10–25 runs. pKa measurements The surface pKa values of LNPs were determined as described previously [34] . Briefly, solutions of 20 mM sodium phosphate, 25 mM citrate, 20 mM ammonium acetate and 150 mM NaCl were titrated to pH values varying by 0.5 from 2.0 to 12.0 and aliquoted into a black 96-well plate. LNPs and 2-( p -toluidinyl)naphthalene-6-sulphonic acid (TNS, Sigma Aldrich) were diluted into these solutions for a final concentration of 20 and 6 μM, respectively. Fluorescence intensity was read on a Tecan M1000 plate reader at an excitation of 322 nm and an emission of 431 nm. pKa values were calculated as the pH corresponding to 50% LNP protonation, assuming minimum and maximum fluorescence values corresponded to zero and 100% protonation, respectively. How to cite this article: Whitehead, K. A. et al. Degradable lipid nanoparticles with predictable in vivo siRNA delivery activity. Nat. Commun. 5:4277 doi: 10.1038/ncomms5277 (2014).